High-performance artificial nitrogen fixation at ambient conditions using a metal-free electrocatalyst Conversion of naturally abundant nitrogen to ammonia is a key (bio)chemical process to sustain life and represents a major challenge in chemistry and biology. Electrochemical reduction is emerging as a sustainable strategy for artificial nitrogen fixation at ambient conditions by tackling the hydrogen- and energy-intensive operations of the Haber–Bosch process. However, it is severely challenged by nitrogen activation and requires efficient catalysts for the nitrogen reduction reaction. Here we report that a boron carbide nanosheet acts as a metal-free catalyst for high-performance electrochemical nitrogen-to-ammonia fixation at ambient conditions. The catalyst can achieve a high ammonia yield of 26.57 μg h –1 mg –1 cat. and a fairly high Faradaic efficiency of 15.95% at –0.75 V versus reversible hydrogen electrode, placing it among the most active aqueous-based nitrogen reduction reaction electrocatalysts. Notably, it also shows high electrochemical stability and excellent selectivity. The catalytic mechanism is assessed using density functional theory calculations. Ammonia (NH 3 ) is an essential building block for manufacturing synthetic chemicals, such as fertilizers, medicaments, dyes, explosives, and resins [1] , [2] , [3] . NH 3 has also received attention as an alternative energy carrier to advance a low-carbon society due to its large hydrogen capacity (17.6 wt%) and high energy density (4.3 kWh h –1 ) [4] . The ever-increasing demand for NH 3 has stimulated significant research interest in artificial nitrogen (N 2 ) fixation [5] , [6] , [7] , [8] , [9] , [10] , [11] , [12] , [13] . Currently, industrial-scale NH 3 production mainly relies on the Haber–Bosch process at high temperature and pressure using N 2 and hydrogen (H 2 ) as feed gases [14] , [15] , [16] . However, this process accounts for ~2% of the worldwide energy use, i.e., 34 GJ ton NH3 –1 and produces a large amount of CO 2 (~2 ton CO2 ton NH3 –1 ) [17] , [18] . In this regard, it is highly imperative to develop lower-energy N 2 -fixation methods, ideally operating at low temperature and pressure. Biological N 2 fixation is catalyzed by nitrogenase at ambient conditions through multiple proton and electron transfer steps, requiring a significant energy input delivered by adenosine triphosphate (ATP) [11] , [19] , [20] , [21] . Encouragingly, electrochemical N 2 reduction using protons and electrons can be powered by renewable energy from solar or wind sources, offering a promising environmentally benign process for sustainable artificial N 2 fixation at room temperature and pressure [22] , [23] . This process, however, is severely challenged by N 2 activation and demands efficient catalysts for the N 2 reduction reaction (NRR) [24] , [25] , [26] . NRR catalysts based on noble metals (e.g., Au [27] , [28] , Ru [29] , Rh [30] ) show favorable activity, but widespread use is hindered by scarcity and high cost. Much attention has thus focused on designing and developing non-noble-metal alternatives but with low Faradaic efficiency (FE), including Fe 2 O 3 -CNT [31] , Fe 3 O 4 [32] , Li + -incorporated PEBCD/C [33] , MoS 2 [34] , (110)-oriented Mo nanofilm [35] , MoO 3 [36] , Mo 2 N [37] , etc. Recently, Lv et al. have reported improved NRR catalytic performance in an amorphous Bi 4 V 2 O 11 -crystalline CeO 2 hybrid (BVC-A) with a high FE of 10.16% and a NH 3 yield that can reach up to 23.21 μg h –1 mg –1 cat. (ref. [38] ). Compared with the catalysts above, metal-free materials offer an obvious advantage of avoiding metal ion release, thereby reducing the environmental impact. N-doped nanocarbon was recently reported for N 2 reduction electrocatalysis with a remarkable NH 3 yield of 23.8 μg h –1 mg –1 cat. , but its FE is only 1.42% [39] . In this context, the idenfication of new metal-free NRR nanocatalysts that simultaneously achieve high NH 3 formation rate and FE is highly desired, which, however, still remains a key challenge. Boron carbide (B 4 C), one of the hardest materials in nature next to diamond and cubic boron nitride, possesses high mechanical strength, (electro)chemical stability, and good electronic conductivity, and much attention has focused on its electrochemical uses as electrode material or catalyst substrate for batteries and fuel cells [40] , [41] , [42] , [43] . Here we report our recent finding that B 4 C nanosheet behaves as a superb metal-free electrocatalyst toward artificial N 2 fixation with excellent selectivity for NH 3 formation under ambient conditions. In 0.1 M hydrochloric acid (HCl), it is capable of achieving an average NH 3 formation rate and a FE as high as 26.57 μg h –1 mg –1 cat. and 15.95% at –0.75 V, respectively, placing it among the most active aqueous-based NRR electrocatalysts. Notably, it also shows high electrochemical stability. In 0.1 M sodium sulfate (Na 2 SO 4 ), the catalyst still exhibits good activity and selectivity with an NH 3 yield of 14.70 μg h –1 mg –1 cat. and a FE of 9.24%. Density functional theory (DFT) calculations suggest that the *NH 2 –*NH 2 →*NH 2 –*NH 3 reaction is the rate-limiting step. Synthesis and characterization of boron carbide nanosheet The B 4 C nanosheet was produced by liquid exfoliation of bulk B 4 C (see Methods for preparation details). As shown in Fig. 1a , the X-ray diffraction (XRD) pattern for B 4 C is highly crystalline with diffraction peaks at 19.7°, 22.0°, 23.5°, 31.9°, 34.9°, 37.8°, 53.5°, 63.7°, and 66.7° that are indexed to the (101), (003), (012), (110), (104), (021), (205), (125), and (220) planes of B 4 C phase (JCPDS No. 35-0798) [44] , respectively. Further characterization by scanning electron microscopy (SEM) and transmission electron microscopy (TEM) confirm the formation of nanosheets after liquid exfoliation, as shown in Supplementary Fig. 1 and Fig. 1b . The higher magnification TEM image (Fig. 1c ) reveals the formation of few-layered B 4 C nanosheet. The high-resolution TEM (HRTEM) image (Fig. 1d ) of such a nanosheet shows well-resolved lattice fringes with an interplanar distance of 0.280 nm indexed to the (110) plane of B 4 C. The corresponding selected area electron diffraction (SAED) pattern (Fig. 1e ) shows well-defined rings indexed to the (012), (110), and (104) planes of B 4 C. X-ray photoelectron spectroscopy (XPS) spectra of B 4 C in C 1 s (Fig. 1f ) and B 1 s (Fig. 1g ) regions are in good agreement with reported results [45] . The peaks in B 1 s are 187.5 eV and 189.1 eV, which can be associated with the B atoms in B−B and B−C bonds, respectively. The peaks of C 1 s spectrum are 284.6 eV (C−C bond), 286.2 eV (C−O bond) and 281.8 eV (C−B bond). The Raman spectroscopy of the B 4 C presents characteristic Raman peaks at 270, 320, 481, 531, 728, 830, 1000, and 1088 cm –1 assigned to crystalline B 4 C (Supplementary Fig. 2 ) [46] . Fig. 1 Structure, morphology, and composition characterizations. a X-ray diffraction (XRD) pattern for B 4 C. b , c Transmisson electron microscopy (TEM) micrograph ( b ) and further magnified TEM images ( c ) for B 4 C nanosheets. d , e High-resolution TEM image ( d ) and selected area electron diffraction (SAED) pattern for one B 4 C nanosheet ( e ). Scale bars, b 1 μm; c 300 nm; d 5 nm; e 5 nm −1 . f , g X-ray photoelectric spectra of B 4 C nanosheets in the B 1 s ( f ) and C 1 s ( g ) regions Full size image Electrocatalytic nitrogen reduction performance The NRR catalytic performance is examined at controllable applied voltages using a three-electrode system comprising of a graphite rod as a counter electrode, Ag/AgCl as a reference electrode and a B 4 C nanosheet-loaded carbon paper electrode (CPE) as a working electrode (B 4 C/CPE; B 4 C nanosheet loading: 0.1 mg cm −2 ). During electrolysis, N 2 gas is bubbled into the cathode, where protons transported from the electrolyte (0.1 M HCl aqueous solution) can react with N 2 on the surface of the catalyst to produce NH 3 . As shown in Fig. 2a , the current of chrono-amperometry curves at different potentials exert good stability. The current density starts high and then decreases to a steady state, which might be ascribed to double layer charging and a result of decreasing local concentration of H + and N 2 near the electrode surface [47] . Fig. 2 Electrocatalytic nitrogen reduction performance. a Chrono-amperometry curves at various potentials in N 2 -saturated 0.1 M HCl. b Ultraviolet-visible (UV-Vis) absorption spectra of the 0.1 M HCl electrolytes stained with indophenol indicator after electrolysis at a series of potentials for 2 h (7200 s). c NH 3 yields and Faradaic efficiencies (FEs) at each given potential in 0.1 M HCl. d Amounts of NH 3 generated with a carbon paper electrode (CPE) and a B 4 C/CPE electrode after 2-h electrolysis at potential of −0.75 V under ambient conditions Full size image To confirm the successful N 2 electroreduction in 0.1 M HCl, the production of both NH 3 and a possible by-product hydrazine (N 2 H 4 ) are spectrophotometrically evaluated after 2-h electrolysis operation by the indophenol blue method [7] and the method of Watt and Chrisp [48] , respectively (the corresponding calibration curves are shown in Supplementary Fig. 3 – 4 ). Figure 2b shows the UV-Vis absorption spectra of electrolyte colored with indophenol indicator at a series of potentials under N 2 bubbling. 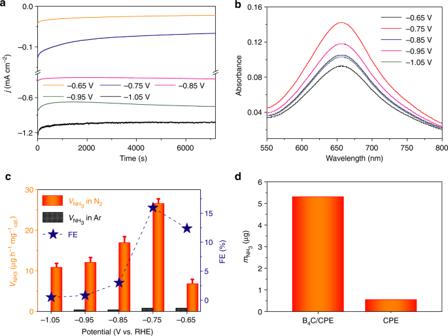Fig. 2 Electrocatalytic nitrogen reduction performance.aChrono-amperometry curves at various potentials in N2-saturated 0.1 M HCl.bUltraviolet-visible (UV-Vis) absorption spectra of the 0.1 M HCl electrolytes stained with indophenol indicator after electrolysis at a series of potentials for 2 h (7200 s).cNH3yields and Faradaic efficiencies (FEs) at each given potential in 0.1 M HCl.dAmounts of NH3generated with a carbon paper electrode (CPE) and a B4C/CPE electrode after 2-h electrolysis at potential of −0.75 V under ambient conditions This detection of NH 3 is concrete and unambiguous proof of NH 3 formation via the electroreduction of N 2 in our B 4 C/CPE platform at potential ranges from −0.65 V to −1.05 V. The average NH 3 yields and corresponding FEs were determined to exemplify the B 4 C nanosheet as an efficient catalyst for the fixation of inert N 2 molecules into highly valuable NH 3 (Fig. 2c ). 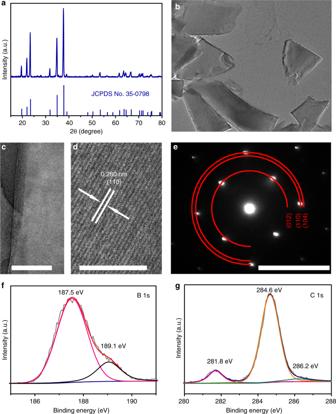As observed, NH 3 yields increase with more negative potential until reaching −0.75 V, where the maximum value of NH 3 yield is calculated as 26.57 μg h –1 mg –1 cat. Fig. 1 Structure, morphology, and composition characterizations.aX-ray diffraction (XRD) pattern for B4C.b,cTransmisson electron microscopy (TEM) micrograph (b) and further magnified TEM images (c) for B4C nanosheets.d,eHigh-resolution TEM image (d) and selected area electron diffraction (SAED) pattern for one B4C nanosheet (e). Scale bars,b1 μm;c300 nm;d5 nm;e5 nm−1.f,gX-ray photoelectric spectra of B4C nanosheets in the B 1s(f) and C 1s(g) regions with a FE of 15.95%, outperforming most reported aqueous-based NRR catalysts at ambient conditions (Supplementary Table 1 ). The NH 3 yield and FE of NRR increase initially (−0.65 V to −0.75 V) and then start to decrease as the potential is negatively shifted to −1.05 V, which is attributed to the FE of the hydrogen evolution reaction that rises slowly (−0.65 to −0.75 V) and then rises rapidly beyond the cathodic polarization potential of −0.75 V (Supplementary Fig. 5 ) [49] . Of note, N 2 H 4 was not detected, indicating this catalyst possesses excellent selectivity for NH 3 formation (Supplementary Fig. 6 ). It is also important to mention that bare CPE has poor electrocatalytic NRR activity (Fig. 2d ), revealing that the B 4 C nanosheet is highly active to catalyze N 2 electroreduction. To verify that the detected NH 3 molecules mainly originate from the electrocatalyzed conversion of N 2 by B 4 C/CPE, control experiments were carried out with an Ar-saturated electrolyte as a function of applied potential and with no potential applied to the electrodes under N 2 gas (open circuit voltage). The corresponding UV-Vis absorption spectra (Supplementary Fig. 7 ) and calculated NH 3 yields (Fig. 2c ) show the presence of a tiny amount of NH 3 that may come from sources of contamination (e.g., laboratory, equipment, membrane). A 15 N isotopic labeling experiment was also performed to verify the N source of the produced NH 3 . As shown in Supplementary Fig. 8 , the standard samples show a triplet coupling for 14 NH 4 + and a doublet coupling for 15 NH 4 + in the 1 H nuclear magnetic resonance ( 1 H NMR) spectra, and the use of 14 N 2 and 15 N 2 as the feeding gas yields 14 NH 4 + and 15 NH 4 + , repsectively. These results provide another piece of evidence to strongly support that NH 3 was produced by B 4 C-catalyzed electroreduction of N 2 . Stability is also a critical parameter of NRR performance for practical applications. Under sustained N 2 gas flow, 30-h electrolysis at a potential of −0.75 V only leads to a slight decrease in current density (Fig. 3a ). After long-term electrolysis, the NH 3 yield for B 4 C/CPE shows only 8% decrease compared with the initial one (Supplementary Fig. 9 ). Furthermore, B 4 C/CPE presents small changes in NH 3 yield and FE during consecutive recycling tests at −0.75 V for 7 times (Fig. 3b ), indicating that high electrocatalytic activity for NRR is maintained very well. The TEM image of a B 4 C nanosheet after long-term electrocatalysis (Supplementary Fig. 10 ) shows almost no obvious change in morphology. XRD analysis (Supplementary Fig. 11 ) and XPS spectra (Supplementary Fig. 12 ) confirm that this catalyst is still B 4 C in nature after NRR. All these results indicate that this catalyst is robust enough to afford NRR electrocatalysis, which may be attributed to the excellent chemical and electrochemical stability of B 4 C in acid and its intrinsic high mechanical strength [42] . Fig. 3 Durability tests. a Time-dependent current density curve and ( b ) recycling test of B 4 C/carbon paper electrode (CPE) at a potential of −0.75 V under ambient conditions Full size image The NRR activity of B 4 C/CPE was also assessed in neutral media (0.1 M Na 2 SO 4 ). Production of NH 3 and the possible by-product (N 2 H 4 ) were evaluated by a spectrophotometry method [31] , [48] . The calibration curves are shown in Supplementary Fig. 13 – 14 . B 4 C/CPE still exhibits excellent selectivity without N 2 H 4 production (Supplementary Fig. 15 ). As shown in Supplementary Fig. 16 – 17 , the NH 3 yield can reach the highest value of 14.70 μg h –1 mg –1 cat. with a FE of 9.24% at potential of −0.75 V. Time-dependent current density curves of B 4 C/CPE for NRR at different potentials suggest excellent stability (Supplementary Fig. 18 ). To identify the active site and atomistic electrocatalytic processes of the NRR on the B 4 C surface, we used the exchange-correlation functional of Perdew, Burke, and Ernzerhof and the dispersion correction method of Grimme (PBE-D) in the framework of DFT to simulate the corresponding electrocatalytic reactions on the B 4 C (110) surface using a periodic slab model (see Methods for details). It is well known that the N 2 adsorption on the catalyst surface is the first step to initialize the NRR and its initial adsorption configuration plays a vital role for subsequent catalytic reactions. Thus, we have first examined the N 2 adsorption on the B 4 C (110) surface. There are two main configurations available for the N 2 adsorption on the B 4 C (110) surface. In the end-on configuration, only one terminal N atom is bonded to the B atom on the B 4 C (110) surface; in the side-on configuration, two terminal N atoms are separately bonded to two vertical B atoms that are located on two adjacent boron clusters (Supplementary Fig. 19 ). The N 2 adsorption potential energies in these two structures are calculated to be 0.65 eV and 0.63 eV at the PBE-D level (free energies: 0.41 eV and 0.34 eV, Supplementary Table 2 ). Since both configurations have similar energy profiles for the electrochemical N 2 fixation reaction on the B 4 C (110) surface, in the following, we have merely focused on discussing the one starting from the end-on configuration. Figure 4 shows our DFT computed energy profiles for the electrocatalytic NRR processes on the B 4 C (110) surface starting from the end-on adsorption structure (optimized structures, Supplementary Fig. 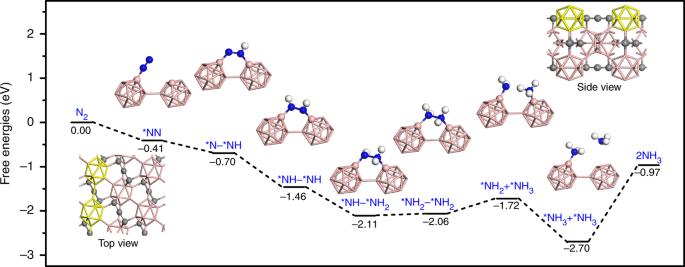Fig. 4 Density functional theory calculations. Density functional theory (DFT) of Perdew, Burke, and Ernzerhof with the dispersion correction method of Grimme (PBE-D) calculated energy profiles for the electrocatalytic N2fixation reaction on the B4C (110) surface starting from the end-on adsorption structure (see optimized structures in Supplementary Fig.20; energy profiles from the side-on adsorption structure in Supplementary Fig.22). Color code: blue, N; rose, B; gray, C; white, H; the asterisk * denotes an adsorption site 20 ). The initial adsorption of molecular nitrogen in this end-on configuration releases 0.41 eV free energy. It can be found that the reaction process from the adsorbed *NN to *NH–*NH 2 species is completely barrierless and releases 1.70 eV free energy at potential of 0.00 V. The following reaction step, i.e., *NH–*NH 2 → *NH 2 –*NH 2 , is also facile because of a small energy gap of 0.05 eV (PBE-D level). Different from the situation of other electrocatalyts, the rate-limiting step of the NRR on the B 4 C (110) surface corresponds to the *NH 2 –*NH 2 → *NH 2 + *NH 3 reaction, which needs to overcome a barrier of 0.34 eV at potential of 0.00 V (i.e., from −2.06 to −1.72 eV). The final electrocatalytic addition reaction of a proton and electron pair on the adsorbed *NH 2 species is barrierless. By contrast, the desorption of the NH 3 molecule, i.e. *NH 3 →NH 3 , demands 1.73 eV free energy. Nevertheless, such a process remains energetically efficient concerning a lot of accumulated free energy in previous reaction processes (2.70 eV at potential of 0.00 V; see Fig. 4 ). Further discussion on the limiting potential of the NRR and the associated energy profile (Supplementary Fig. 21 ) can be found in Supplementary information. Finally, the energy profiles for the electrocatalytic processes starting from the side-on adsorption structure are similar to those from the end-on one (Supplementary Fig. 22 ). Fig. 4 Density functional theory calculations. Density functional theory (DFT) of Perdew, Burke, and Ernzerhof with the dispersion correction method of Grimme (PBE-D) calculated energy profiles for the electrocatalytic N 2 fixation reaction on the B 4 C (110) surface starting from the end-on adsorption structure (see optimized structures in Supplementary Fig. 20 ; energy profiles from the side-on adsorption structure in Supplementary Fig. 22 ). Color code: blue, N; rose, B; gray, C; white, H; the asterisk * denotes an adsorption site Full size image In summary, a B 4 C nanosheet has been experimentally proven as a superior metal-free electrocatalyst for artificial N 2 fixation to NH 3 with excellent selectivity at room temperature and ambient pressure. This catalyst achieves a high NH 3 yield of 26.57 µg h –1 mg –1 cat. and a high FE of 15.95% at a potential of −0.75 V in 0.1 M HCl, with high electrochemical stability. Impressively, B 4 C/CPE still exhibits good NRR activity in neutral media. Further DFT calculations reveal that the *NH 2 –*NH 2 →*NH 2 –*NH 3 reaction is the rate-limiting step. This study not only provides an attractive metal-free electrocatalyst material for NH 3 synthesis, but also opens up an exciting new avenue to the rational design of B 4 C-based nanocatalysts with enhanced performance for N 2 -fixation applications. Sample preparation Commercial bulk B 4 C was purchased from Aladdin Ltd. (Shanghai, China). All reagents were analytical reagent grade without further purification. The water used throughout all experiments was purified through a Millipore system. A total of 1 g bulk B 4 C was dispersed in 10 mL ethanol and stripped by ultrasonic cell disruptor for 1 h. Subsequently, the resulting dispersion was centrifuged for 10 min at 3000 rpm and the supernatant containing B 4 C nanosheet was decanted gently. Next, 710 µL of the obtained solution was added into 250 µL H 2 O containing 40 µL of 5 wt% Nafion and sonicated for 1 h to form a homogeneous ink. Then, 50 µL of the dispersion was loaded onto a carbon paper electrode with area of 1 × 1 cm 2 and dried under ambient conditions, the catalyst loading mass is 0.1 mg cm –2 . Characterization XRD pattern was recorded using a LabX XRD-6100 X-ray diffractometer, with a Cu Kα radiation (40 kV, 30 mA) of wavelength 0.154 nm (SHIMADZU, Japan). The structures of the samples were determined by TEM images on a HITACHI H-8100 electron microscopy (Hitachi, Tokyo, Japan) operated at 200 kV. SEM image was obtained on a Hitachi S-4800 field emission scanning electron microscope at an accelerating voltage of 20 kV. XPS measurements were performed on an ESCALABMK II X-ray photoelectron spectrometer using Mg as the exciting source. The absorbance data of spectrophotometer were measured on SHIMADZU UV-1800 UV-Vis spectrophotometer. A gas chromatograph (SHIMADZU, GC-2014C) equipped with MolSieve 5A column and Ar carrier gas was used for H 2 quantifications. Gas-phase product was sampled every 1000 s using a gas-tight syringe (Hamilton). 1 H NMR spectra were collected on a superconducting-magnet NMR spectrometer (Bruker AVANCE III HD 500 MHz) and dimethyl sulphoxide was used as an internal to calibrate the chemical shifts in the spectra. Electrocatalytic nitrogen reduction measurements The reduction of N 2 gas (99.99%) was carried out in a two-compartment cell under ambient condition, which was separated by Nafion 211 membrane. The membrane was protonated by first boiling in ultrapure water for 1 h and treating in H 2 O 2 (5%) aqueous solution at 80 °C for another 1 h, respectively. And then, the membrane was treaded in 0.5 M H 2 SO 4 for 3 h at 80 °C and finally in water for 6 h. The electrochemical experiments were carried out with an electrochemical workstation (CHI 660E). The potentials reported in this work were converted to reversible hydrogen electrode (RHE) scale via calibration with the following equation: E (vs. RHE) = E (vs. Ag/AgCl) + 0.256 V and the presented current density was normalized to the geometric surface area. For electrochemical N 2 reduction, chrono-amperometry tests were conducted in N 2 -saturated 0.1 M HCl solution (the HCl electrolyte was purged with N 2 for 30 min before the measurement). Quantification of ammonia When tested in 0.1 M HCl, the concentration of NH 3 produced was spectrophotometrically determined by the indophenol blue method [7] . Typically, 2 mL HCl electrolyte was taken from the cathodic chamber, and then 2 mL of 1 M NaOH solution containing 5% salicylic acid and 5% sodium citrate was added into this solution. Subsequently, 1 mL of 0.05 M NaClO and 0.2 mL of 1% C 5 FeN 6 Na 2 O·2H 2 O were add into the above solution. After standing at room temperature for 2 h, the UV-Vis absorption spectrum was measured at a wavelength of 655 nm. The concentration-absorbance curves were calibrated using standard NH 3 solution (Supplementary Fig. 3 ) with a series of concentrations. The fitting curve ( y = 1.130 x + 0.078, R 2 = 0.999) shows good linear relation of absorbance value with NH 3 concentration by three times independent calibrations. When tested in 0.1 M Na 2 SO 4 , the NH 3 concentration was measured by a spectrophotometry method [31] . In detail, 4 mL of post-tested solution was removed from the cathodic chamber. Then, 50 μL of oxidizing solution (NaClO ( ρ Cl = ~4–4.9) and 0.75 M NaOH), 500 µL of coloring solution (0.4 M C 7 H 5 O 3 Na and 0.32 M NaOH) and 50 µL of catalyst solution (0.1 g Na 2 [Fe(CN) 5 NO] 2H 2 O diluted to 10 mL with deionized water) were added sequentially to the sample solution. After standing at 25 °C for 1 h, the UV-Vis absorption spectra were performed. The concentration of indophenol blue was determined using the absorbance at a wavelength of 655 nm. The concentration-absorbance curve was calibrated using standard NH 3 solution with a series of concentrations. The fitting curve ( y = 0.753 x + 0.026, R 2 = 0.999) shows good linear relation of absorbance value with NH 3 concentration by three times independent calibrations (Supplementary Fig. 13 ). Quantification of hydrazine The amount of N 2 H 4 present in the electrolyte was estimated by the method of Watt and Chrisp [48] . A mixed solution of 5.99 g C 9 H 11 NO, 30 mL HCl, and 300 mL ethanol was used as a color reagent. Calibration curve was plotted as follow: first, preparing a series of standard solutions; second, adding 5 mL above prepared color reagent and stirring 20 min at room temperature; finally, the absorbance of the resulting solution was measured at 455 nm, and the yields of N 2 H 4 were estimated from a standard curve using 5 mL residual electrolyte and 5 mL color reagent. Absolute calibration of this method was achieved using N 2 H 4 solutions of known concentration as standards, and the fitting curve shows good linear relation of absorbance with N 2 H 4 concentration in 0.1 M HCl (Supplementary Fig. 4 , y = 0.545 x + 0.031, R 2 = 0.999) and 0.1 M N 2 SO 4 (Supplementary Fig. 14 , y = 1.199 x + 0.051, R 2 = 0.999) by three times independent calibrations. Calculation of the Faradaic efficiency and yield The FE for N 2 reduction was defined as the amount of electric charge used for synthesizing NH 3 divided the total charge passed through the electrodes during the electrolysis. The total amount of NH 3 produced was measured using colorimetric methods. Assuming three electrons were needed to produce one NH 3 molecule, the FE could be calculated as follows: 
    FE = 3 × F × C_NH_3× V/17 × Q. (1) The rate of NH 3 formation \(({v_{{\mathrm{NH}}_3}})\) was calculated using the following equation: 
    v_NH_3 = C_NH_3× V/t ×m_cat..
 (2) where F is the Faraday constant, \({\rm C}_{{\rm NH}_3}\) is the measured NH 3 concentration, V is the volume of the HCl electrolyte for NH 3 collection, t is the reduction time and m cat . is the catalyst loading mass. FE for H 2 was calculated according to following equation: 
    FE = 2 ×F×n/Q,
 (3) where F is the Faraday constant; n is the actually produced H 2 (mol), and Q is the quantity of applied electricity. Calculation details All DFT calculations are performed using the DMol [3] module implemented in the Material Studio 8.0 package [50] , [51] . The generalized gradient approximation (GGA) with the PBE exchange-correlation functional is employed [52] . The empirical dispersion correction proposed by Grimme is used to consider weak van der Waals interaction [53] . 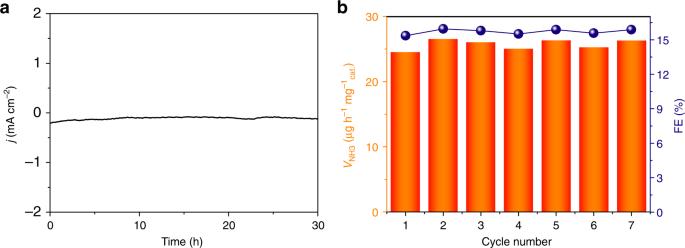The build-in double numerical plus polarization (DNP) basis set is used to expand the electronic wavefunction. Fig. 3 Durability tests.aTime-dependent current density curve and (b) recycling test of B4C/carbon paper electrode (CPE) at a potential of −0.75 V under ambient conditions A Monkhorst-Pack k-point grids of 2 × 1 × 1 are used (see Supplementary Table 3 for benchmark). Self-consistent field (SCF) calculations are performed with a convergence criterion of 10 −6 au on the total energy and electronic computations. Since the bulk water layer only slightly stabilizes the NRR intermediates [54] , we have therefore adopted the conductor-like screening model (COSMO) to simulate solvent effects [55] . A three-layer 1 × 2 periodic slab model is used to represent the B 4 C (110) surface that is observed in our HRTEM image (see Supplementary Table 4 for benchmark). A 15 Å vacuum layer is used between the two neighboring slabs to avoid artificial interaction. In geometric optimizations, all atoms except those in the bottom layer are fully relaxed. The adsorption energy (E ads ) of species on the B 4 C (110) surface is defined as: 
    E_ads = E_slab + E_mol - E_slab/mol,
 (4) where E slab and E mol are the energies of the isolated slab and species, respectively; and E slab/mol is the energy of the species-adsorbed slab system. The NRR process includes six net coupled proton and electron transfer (CPET) steps (N 2 + 6H + + 6e − → 2NH 3 ). Based on previous theoretical studies [54] , gaseous hydrogen is used as the source of protons to simulate the reaction at the anode, i.e., H 2 ↔ 2H + + 2e − . Each CPET step includes the transfer of a proton coupled with an electron from solution to an adsorbed species on the B 4 C (110) surface. For each fundamental step, the Gibbs free energy change (ΔG) is calculated based on the standard hydrogen electrode (SHE) model proposed by Nørskov et al. [56] , [57] , [58] in which the chemical potential of a proton-coupled-electron pair i.e., µ(H + ) + µ(e − ) is equal to half of the chemical potential of gaseous hydrogen i.e., 1/2 µ(H 2 ) at a potential of 0 V. Accordingly, the ΔG value can be obtained as follows: 
    Δ G = Δ E + Δ ZPE - TΔ S + Δ G_U + Δ G_pH,
 (5) where ΔE is the electronic energy difference, ΔZPE is the change in zero-point energies, T is the temperature ( T = 298.15 K), and ΔS is the change of entropy. ΔG U is the free energy contribution connected to electrode potential U. ΔG pH is the H + free energy correction by the concentration. It is calculated through ΔG pH = 2.303 × k B T × pH where k B is the Boltzmann constant and the value of pH is assumed to be zero in this work. It can be found that the free energy change of each elementary step is increased as the pH value increases. The zero-point energies and entropies of the NRR species are determined from the vibrational frequencies in which only the adsorbed species’ vibrational modes are computed explicitly and the B 4 C (110) surface is fixed. The entropies and vibrational frequencies of molecules in the gas phase are taken from the NIST database. [ http://cccbdb.nist.gov/ ] Data availability The data described in this paper are available from the authors upon reasonable request.